Relative comparisons of call parameters enable auditory grouping in frogs Whereas many studies on mate choice have measured the relative attractiveness of acoustic sexual signals, there is little understanding of another critical process: grouping and assigning the signals to their sources. For female túngara frogs, assigning the distinct components of male calls to the correct source is a challenge because males sing in aggregations, producing overlapping calls that lead to perceptual errors analogous to those of the 'cocktail party problem'. Here we show that for presentation of >2 call components, however, subjects are more likely to group the two components with the smallest relative differences in call parameters, including relative spatial separation (a primitive acoustic cue) and relative similarity to the species-specific call sequence (a schema-based cue). Thus, like humans, the cognitive rules for the perception of auditory groups amidst multiple sound sources include the use of relative comparisons, a flexible strategy for dynamic acoustic environments. Auditory object formation involves sorting sounds into groups and assigning them to their correct sources [1] , [2] , [3] . Object formation is complicated by the fact that sounds from different sources combine linearly and arrive at a receiver as a single complex wave which is not source specific, meaning groups and source assignment must be 'deduced' [4] , [5] , [6] , [7] . Thus, during acoustic communication [8] , perception of information and identification of its sender are inherently linked to how receivers make such deductions. The auditory system often accomplishes this by deconstructing the complex wave into its individual components, a result of processing so called 'primitive' or 'general purpose' acoustic cues (for example, temporal, spectral, spatial, and amplitude parameters) [3] , [4] , [7] , [9] . Correct grouping and source assignment result from the ability to compare within and between these cues, a process made more difficult when there are multiple sources producing similar sounds. Using an approach most often applied with humans, this study determines how mate-searching female frogs deduce the source of complex male signals in breeding aggregations on the rain forest floor. Tests of object formation often measure the cue or acoustic parameter values that elicit grouping within, but not beyond a certain boundary [10] , [11] , [12] , [13] , [14] . Under conditions in which multiple cues overlap, however, absolute boundaries may not explain all perceptual grouping, as listeners may employ a relative strategy in which objects are formed by grouping stimuli with the most similar acoustic parameters and excluding those more distinct. Indeed, in humans variations of the streaming paradigm have shown that groups are not based on absolute tone differences, but result from relative comparisons among the tones available for grouping. For example, O'Conner and Sutter [15] presented an ascending series of tones that, without background sounds, elicits perception of a single auditory object (that is, the target). If a sequence of background tones is added before and after the target sequence two groups are formed, one of which includes portions of the target that are perceptually captured into the background depending on target-background frequency separation [16] . Thus, the addition of the background 'breaks' the perceptual group that would otherwise be formed in isolation. Taken together with the fact that a complex grouping response-function emerges when the frequency separation between the target tones is also varied, it leads to the conclusion that relative (not absolute) frequency separation can determine the auditory stream [3] , [11] . In addition to primitive cues, object formation is also affected by experience or internal state [6] , [11] , [17] , [18] . These are components of schema-driven object formation, in which the probability of grouping varies with a stimulus' similarity to stored information, such as an innate or learned (for example, instructed) template [7] , [11] . With respect to communication sounds, such a strategy is known from research on human speech [5] , [6] , [9] , [19] . Thus, perceptual groups based on relative comparisons may not be limited to the relative differences in primitive cues, as similarity to schematic templates such as species-specific signal patterns could also be used to deduce auditory objects. The wealth of data on humans notwithstanding, the challenge of object formation is not restricted to our own species. Various species across disparate taxa must also identify and locate complex acoustic signals in multi-source environments [20] , [21] , [22] . Indeed, several groups of animals produce acoustically complex mating calls in multi-male choruses. As with humans during the 'cocktail party problem' [23] , females attending to male choruses must correctly identify and group these overlapping sounds to choose an appropriate mate [24] , [25] , [26] , [27] , [28] . Understanding how females perform this task is critical for evaluating the underlying mechanisms of mate choice and how those mechanisms (and the signals) evolve. Furthermore, this understanding also informs us as to the degree of convergence/divergence in humans and other animals in responding to this challenge. Using female túngara frogs ( Physalaemus pustulosus ), this study tested the hypothesis that auditory grouping of call components results from the comparison of relative spatial (primitive) and call sequence (schema) cues. In multi-male choruses males produce complex calls consisting of two components: the frequency modulated 'whine', which is necessary and sufficient to elicit phonotaxis; followed by 0–7 broadband 'chucks'. Chucks are never produced alone and can only follow a whine due to male vocal anatomy [29] , creating a schema-based cue for whine-chuck grouping. Farris et al . [30] , [31] showed that these two call components are perceptually distinct, as the whine is used in both 'what and where' decisions, and the chuck is only used in 'where' decisions. Important to this study is that phonotaxis to a chuck is contingent on the presentation of a whine [30] , [31] . This combination sensitivity, in part, reveals auditory grouping of the whine and chuck. Previous tests of whine-chuck grouping have shown that absolute spatial and temporal differences have a limited effect (for example, grouping up to 135° whine-chuck separation and for non-natural whine-chuck sequences) and predict that in a dense male chorus whines and chucks from different sources could be incorrectly grouped [30] , [31] . The stimuli in previous tests, however, used only two call components, a single whine and a single chuck. Thus, in this study we determine if such poor grouping acuity would be eliminated in a multi-source (>2 sources) environment by testing whether object formation results from comparisons between available call components: we test the hypothesis that components with the smallest relative differences are more likely to be grouped [15] . Control stimuli As with our previous work [30] , [31] , responses to control stimuli confirm that the whine is necessary and sufficient to elicit and direct phonotaxis ( Fig. 1 ). Data show that exit angles are non-random and localized to the position of the whine ( Fig. 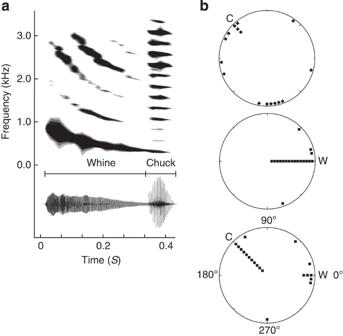Figure 1:Túngara frog call components and conditional response to the chuck. (a) Spectrogram and time waveform of male call. (b) Demonstration of auditory grouping of a single whine and chuck. Squares are the exit angles from the circular arena for individual females. (Top) Responses to the chuck alone are not oriented. (Middle) Whines alone are necessary and sufficient to elicit directed phonotaxis. (Bottom) When a whine and chuck (with normal timing) are spatially separated up to 135°, females move to the chuck, indicating these two stimuli are perceived as a single object at the location of the chuck. Data are from a previous study30. Polar coordinates are the same in all figures and tables. C, location of a chuck; W, location of a whine. 2 ; Table 1 ). New to this study is the control showing that the presentation of two chucks without a whine elicits the same response as that for the presentation one chuck [30] , [31] . First, chucks often do not elicit a response ( Table 1 ). Second, circular analysis shows that if responses do occur, their direction is randomly distributed. Third, when compared to the categorical responses to a single chuck in our two previous studies [30] , [31] (that is, 11.6% of females are expected to exit the arena within 10° of any chuck), the percentage of responses to either chuck of the 2-chucks stimulus was not significantly different ( Fig. 2 ; Table 1 ). Thus, the failure of the two chucks to elicit a directed response maintains the critical control for concluding auditory grouping of the complex call components: phonotaxis to any chuck occurs only in the presence of the whine. Figure 1: Túngara frog call components and conditional response to the chuck . ( a ) Spectrogram and time waveform of male call. ( b ) Demonstration of auditory grouping of a single whine and chuck. Squares are the exit angles from the circular arena for individual females. (Top) Responses to the chuck alone are not oriented. (Middle) Whines alone are necessary and sufficient to elicit directed phonotaxis. (Bottom) When a whine and chuck (with normal timing) are spatially separated up to 135°, females move to the chuck, indicating these two stimuli are perceived as a single object at the location of the chuck. Data are from a previous study [30] . Polar coordinates are the same in all figures and tables. C, location of a chuck; W, location of a whine. 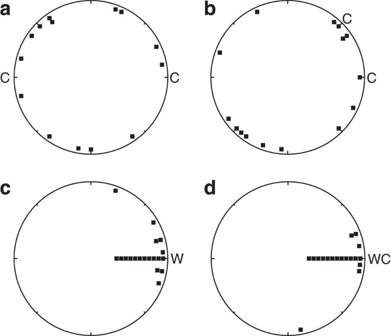Figure 2: Exit angles for control stimuli. (a) Two chucks with 180° spatial separation; (b) Two chucks with 45° spatial separation; (c) Whine presented alone; (d) Whine-chuck with normal timing and 0° spatial separation. C, chuck; W, whine. Full size image Figure 2: Exit angles for control stimuli. ( a ) Two chucks with 180° spatial separation; ( b ) Two chucks with 45° spatial separation; ( c ) Whine presented alone; ( d ) Whine-chuck with normal timing and 0° spatial separation. C, chuck; W, whine. Full size image Table 1 Analysis of phonotaxis direction for a whine or chucks alone or in natural combination. Full size table Spatial separation on same side of the whine Responses to broadcasts of a whine and a pair of chucks with different relative whine-chuck separations show that grouping is more likely for the chuck closest to the whine ( Fig. 3 ; Table 2 ). When the closest chuck has a 0° spatial separation relative to the whine, exit angles were non-randomly distributed and the mean exit angles did not differ from 0°. Furthermore, the presence of the second, more spatially separated chuck did not alter responses when compared to those for a single whine and chuck at 0° spatial separation ( Fig. 3a–d ; Table 2 ). Confounded in this stimulus set, however, is the fact that the chuck closest to the whine is broadcast from the same position of the whine, meaning the design can not distinguish conditional responses to the closest chuck from those to the whine. Using broadcasts of two spatially separated chucks with the closest at 45° (re. whine) revealed the same response, however. First, control data with two chucks of equal whine-chuck separation show that 16/24 trials exhibited grouping. There was no bias to either chuck, as equal separation elicits equal probability of being grouped with the whine (7/24 vs 9/24; P =0.38; Fig. 3e ). When one chuck is separated farther, however, data show strong grouping of the closest chuck: the response is not random and the mean exit angle is not different from 45°. Furthermore, the mean exit angle is nearly identical to that for a single whine-chuck stimulus at 45° spatial separation ( Fig. 3f–h ; Table 2 ). This means that grouping of the closest chuck is categorical, as there is no evidence that females averaged the position of the two chucks. 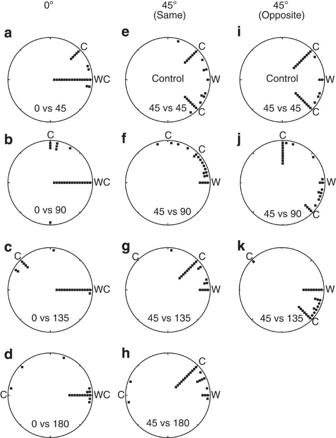Figure 3: Exit angles in response to a whine presented with two competing chucks. Each chuck has a natural timing but at varying whine-chuck separations. (a–d) Closest chuck has 0° whine-chuck separation. (f–h) Closest chuck is 45° from the whine, with both chucks on same side of whine. (i–k) Closest chuck is 45° from the whine, but on opposite sides. (e, i) Controls with chucks at 45° on each side of the whine were run for each experiment. C, chuck; W, whine. Figure 3: Exit angles in response to a whine presented with two competing chucks. Each chuck has a natural timing but at varying whine-chuck separations. ( a – d ) Closest chuck has 0° whine-chuck separation. ( f–h ) Closest chuck is 45° from the whine, with both chucks on same side of whine. ( i–k ) Closest chuck is 45° from the whine, but on opposite sides. ( e, i ) Controls with chucks at 45° on each side of the whine were run for each experiment. C, chuck; W, whine. Full size image Table 2 Analysis of phonotaxis direction for a whine with two spatially separated chucks in natural temporal sequence. Full size table Spatial separation on opposite sides of the whine The previous experiments created whine-chuck separations in one hemisphere of the circular arena. This means that when facing the whine the two chucks would be lateralized to the same side of the frog, potentially engaging different mechanisms for assessing spatial coherence than if the chucks were lateralized to different sides. Thus, we tested whether stimulus orientation affects spatial grouping such that the two chucks are now on opposite sides of the whine. Control data for equal separation ( Fig. 3i ; 45° vs 45°) again showed no bias in grouping responses to either of the chucks (10/25 vs 11/25; P =0.5). For different separations, only the 45° vs 135° chuck separation matched the response of the same-side stimuli above, as the mean exit angle was significantly localized at the closest chuck and the distribution was not different from that for a whine and single chuck at 45° ( Fig. 3k ; Table 2 ). Grouping of the chuck closest to the whine, however, did not hold when the relative spatial separations of the two chucks were 45° and 90° on opposite sides of the whine ( Fig. 3j ; Table 2 ), as responses were more similar to the 45° vs 45° control. Masking verses grouping spatial acuity The results above suggest that while grouping whines and chucks, spatial resolution during presentation of a pair of chucks is more acute (45°) than that for grouping a single chuck (≤135°) [30] , [31] . Also, grouping responses to multi-chuck stimuli appeared categorical or limited to one chuck at a time, as the responses shown in Figure 3 reveal that exit angles are not located at a position that is an average of the two chucks. Taken together, these data generate the hypothesis that increased spatial resolution during the multi-chuck stimulus prevents detection of the non-grouped chuck. To test this, the grouping experimental paradigm is combined with that of spatial masking by presenting a whine, a single chuck and a burst of white noise with the same envelope and temporal parameters of the chuck (that is, replacing the second chuck). The experiment tested if during whine-chuck grouping a third, non-grouped, spatially separated stimulus is indeed detected by observing whether the noise burst could mask the chuck. A premise of this experiment is that the noise is a masker and does not elicit a phonotactic or grouping response on its own. Thus, control broadcasts first established that a broadband noise with same envelope structure of a chuck is not grouped ( Fig. 4 ). Like chucks broadcast alone, the noise alone does not elicit phonotaxis and exit angles are not significantly different from random (r=0.16; P =0.652). When the noise is presented with the whine (90° spatial separation), although there is a significant shift in mean exit angle away from that generated from presenting a whine alone (mean angle: whine 94.3° vs whine-noise 60.8°; F=15.7; P <0.0003; Fig. 4 ), this shift is significantly less than that for a grouped chuck, as the whine-chuck response is significantly closer to the chuck position (mean angle: whine-noise 60.8° vs whine-chuck 28.0°; F=9.0; P <0.005). Furthermore, in categorical analysis, the number of direct responses to the noise (±10°) broadcast with the whine is not significantly different from that when the noise is broadcast alone (whine-noise 4/25 vs noise alone 3/25; P =0.5; Fig. 4 ). And, this number is significantly less than that measured for attraction to a chuck broadcast with a whine (whine-noise 4/25 vs whine-chuck 16/25; P <0.0007). Thus, the broadcast of a spatially separated noise at the natural temporal position of a chuck does not elicit the grouping response. These data allow for the noise to be used as a masker. 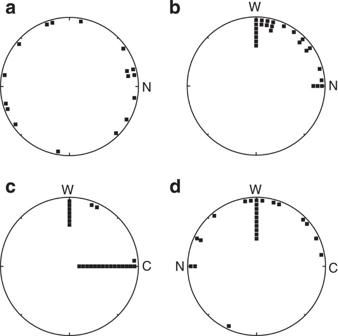Figure 4: Spatial resolution for masking and grouping are not the same. (a) Broadband noise (N) with the same envelope of the chuck does not evoke orientation by females. (b) Noise broadcast with a whine shifts response orientation, but does not elicit grouping response like that for a whine-chuck (c). (d) Noise broadcast simultaneously with a naturally timed chuck prevents grouping at 180° spatial separation. C, chuck; W, whine. Figure 4: Spatial resolution for masking and grouping are not the same. ( a ) Broadband noise (N) with the same envelope of the chuck does not evoke orientation by females. ( b ) Noise broadcast with a whine shifts response orientation, but does not elicit grouping response like that for a whine-chuck ( c ). ( d ) Noise broadcast simultaneously with a naturally timed chuck prevents grouping at 180° spatial separation. C, chuck; W, whine. Full size image When the noise is presented simultaneously with the chuck, each at 90° from the whine and 180° from each other, the chuck is no longer grouped ( Fig. 4 ). Direct responses to the chuck are significantly reduced (whine-chuck 16/25 vs whine-chuck+noise 1/25; P <0.00005) and the mean exit angle is nearly identical to that for the whine alone (whine 94.3° vs whine-chuck+noise 93.5°; F=0.0043; P =0.948). In addition to these analyses showing the effect on grouping by adding noise to a single whine-chuck stimulus ( Fig. 4 ), the effect is also illustrated when comparing responses to a multi-chuck stimulus ( Fig. 4d vs Fig. 5b ). Thus, the response is consistent with masking. And, although we found a 45° resolution between multiple chucks during the grouping response ( Fig. 3 ), this resolution does not appear to be based on limits of spatial unmasking, which was evident for our only chuck-noise separation at 180°. Note that no other (smaller) separations were tested because acuity was determined at the largest angle. 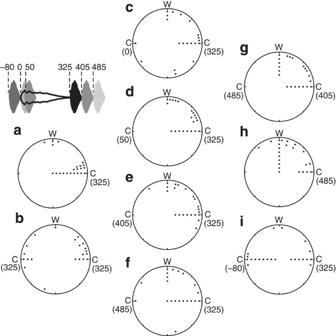Figure 5: The effects of relative whine-chuck sequence on grouping. Squares are exit angles in response to two competing chucks with the same separations (90° re. whine), but different timings (in parentheses, in ms relative to whine onset). Natural chuck timing is 325 ms. Letter for each plot (a–i) corresponds to stimulus designation inTable 3. Upper left is a diagram of the whine (open shape; onset time is 0 ms) and different chuck onset times to show the extent of temporal overlap. Figure 5: The effects of relative whine-chuck sequence on grouping. Squares are exit angles in response to two competing chucks with the same separations (90° re. whine), but different timings (in parentheses, in ms relative to whine onset). Natural chuck timing is 325 ms. Letter for each plot ( a – i ) corresponds to stimulus designation in Table 3 . Upper left is a diagram of the whine (open shape; onset time is 0 ms) and different chuck onset times to show the extent of temporal overlap. Full size image Schema-based grouping The morphologically constrained whine-then-chuck sequence ( Fig. 1 ) provides a cue for grouping and source assignment. Because the cue is based on stored information on the part of the receiver and not on source acoustics, results here address whether grouping in túngara frogs is schema-driven. Following the letters designating stimuli in Table 3 , control stimuli (stims. a, b ) first reconfirm that a naturally timed chuck at 90° spatial separation from the whine is grouped ( Table 3 ; Fig. 5a,b ). The addition of a second simultaneous chuck (equal separation, opposite side of the arena) showed that there is no bias in the arena: either chuck may be grouped, which is reflected in the bimodal distribution of the exit angles and their high dispersion (r). Also, the distribution is not different from random (stim. b ; Fig. 5b ). Table 3 Analysis of phonotaxis direction for a whine with two chucks at equal separation, but timed differently relative to the onset of the whine. Full size table In four of the stimulus conditions, the grouping response favored the chuck timed to the natural sequence. First, when the natural-timed chuck is broadcast with chucks that could not be produced by single males because they overlap the whine (stims. c, d ; Fig. 5c,d ), the mean exit angles are localized at the natural-timed chuck and the response distributions do not differ from that for a whine followed by a single natural-timed chuck (stim. a , Fig. 5a vs c,d ). Failure to group overlapping chucks is not based on a 'go to the last chuck' rule, however, as the natural-timed chuck is also more likely to be grouped than those that follow it (stims. e, f ). Unlike the chucks overlapping the whine, the chucks following the natural-timed chuck could be produced by a male. Stimulus condition g tests whether the decision rule is particular to the natural temporal position or just chucks timed closest to it ( Table 3 ). Here, two chucks were presented which could be produced by a male, but neither is timed in the natural position of a single chuck: both are delayed and occupy times when a male would produce second and third chucks. The mean exit angle was not different from the speaker broadcasting the chuck timed closest to natural sequence (that is, the position of the 405 ms onset chuck; Fig. 5g ), which is consistent with the hypothesis that grouping favors chucks closest to the natural time. However, the responses were significantly less directed to that chuck compared to the response to the naturally timed (325 ms onset) chuck presented alone with a whine ( P =0.03, Table 3 ). This suggests an importance of the natural timing window. Furthermore, the failure of the 405 ms onset chuck to completely match responses to a natural-timed chuck occurred even though the last chuck (485 ms onset) did not elicit the same grouping response as the single chuck control (stim. h , Fig. 5h ). Taken together the data suggest that under these stimulus conditions the natural time of a first chuck is weighted more heavily during grouping. It is important to note that there was one striking exception to the dominance of the whine-chuck natural sequence, however. When a chuck precedes the whine, there is no longer significant grouping of the natural sequenced chuck (stim. i , Fig 5i ), as responses are nearly identical to those in control stimulus condition b , with both chucks eliciting grouping ( Table 3 ; Fig. 5 ). With respect to spatial cues, a general similarity in both humans and frogs is that simple auditory spatial resolution is characterized by greater acuity than that used in grouping. In humans, for example, grouping can occur over larger stimulus separations (180°) [9] , [23] , [32] , [33] than the minimum audible angle [34] . Indeed, the weakness of spatial or binaural cues in grouping is revealed by the fact that other cues can override them [35] , [36] , [37] , [38] , [39] . Likewise in frogs, assays of behavior, ear biomechanics, and neurophysiology show that auditory spatial resolution varies with source separations of 90° (ref. 27 ) or much less [40] , [41] , [42] , [43] . In contrast, during sequential pattern recognition similar to auditory streaming, songs may still be grouped or combined when separated by 120–180° (refs 44 , 45 ). Our previous data in P. pustulosus are consistent with this trend, as a single whine and chuck may be grouped over 135° (refs 30 , 31 ) ( Fig. 1 ). Our present study (and data from humans and other frogs) shows, however, that use of spatial cues in grouping is not necessarily weak, in that acuity may be stimulus dependent [9] , [11] , [15] , [32] . For example, whereas segregation of sound sequences by some treefrogs is tolerant of large separations, Bee [46] recently showed that in the context of processing simultaneous sounds, separation of call components by <10° can reduce attractiveness. This difference in spatial acuity between simultaneous and sequential tasks is consistent with that exhibited by humans [47] . Our study adds another stimulus context to such results showing greater acuity in grouping. Importantly, we show that for sounds that would otherwise be grouped over wide spatial separations on their own, greater spatial acuity is revealed with the addition of more sources: use of relative separation for grouping occurs over 45° compared to 135° for a single whine and chuck [30] , [31] . But this greater acuity is limited to certain conditions and stimuli. First, greater spatial acuity during grouping is not uniform for different stimulus orientations. Acuity is reduced (that is, more separation is required for grouping) when chucks are on either side of a whine as opposed to the same side. Second, acuity is limited to the addition of more chucks and not noise, which produced masking over the largest possible separation (180°). The results are important not only for the reduction in acuity, but also because they reveal a strategy that is not based on absolute processing criteria. That is, use of spatial cues in grouping appears flexible. Often, studies of spatial effects on grouping test the extent to which spatial separation still allows for grouping. For example, the spatial separation of a component or set of components in a multi component stimulus is increased until it 'pops out' or is perceived as a separate set of objects. Here, we test a special case where a subject is given a stimulus in which all components are within the spatial separation for grouping. The subject is then asked whether there is equal likelihood of grouping as a function of relative separation. This new context of relative comparisons notwithstanding, our data further demonstrate the stimulus dependence of spatial grouping by showing that responses vary with stimulus orientation and the presence of a masker. Thus, four stimulus contexts are now known to affect spatial acuity when grouping whines and chucks: separation, relative separation, orientation and the presence of a masker. Perception of auditory objects may be based on stored information that is comprised of numerous auditory attributes [6] . Although in túngara frogs there is (so far) no evidence that grouping varies with instructed or learned attributes, there are a plethora of data showing that stored information is employed to evaluate sound. Several studies have shown, for example, that both gross and fine FM characteristics of the whine enable call recognition and conspecific versus heterospecific discrimination [48] , [49] ; working memory varies with signal complexity [50] ; and, whines and chucks are processed differently in recognition and location decisions [30] , [31] . Prior to this study, however, tests of call recognition, preference or grouping of a single whine and chuck revealed little evidence for the use of call sequence in phonotactic decisions [31] , [51] . We now show that information contained in the call sequence can be used to determine call sources when multiple sources are presented. In particular, in all but one case the data implicate a receiver strategy that includes information regarding the production of the whine and chuck to determine their source. That is, chucks occurring at times that are either impossible or less likely to be produced by a single male are not grouped with the whine when a natural-timed chuck is present. For example, chucks overlapping the onset of the whine, although grouped when presented as a single chuck with a whine, are no longer grouped in favor of a second chuck that is timed to the natural sequence. There are no source-specific acoustic reasons for this strategy (for example, location, harmonic relationship, etc. ), leading to the conclusion of schema-based grouping that uses relative comparisons. Our data show that there is variance in this strategy, however, as grouping of a chuck preceding the onset of the whine is as likely as a chuck following the whine in the natural sequence. This exception could be explained if single males used 100% duty cycle to produce a series of calls, placing the chuck from a previous call just before the whine of a subsequent call. This is unlikely, however, as call period is approximately 1.5 s too long [52] . Thus, failure to bias grouping to the natural sequence in this case could still lead to whine-chuck grouping errors in a chorus. Such inaccurate grouping could be a result of preferences for particular male traits, however. Although studied in a preference rather than grouping paradigm, there is evidence that changes in the relative timing of stimuli can alter strong preferences for particular call attributes. For example, in Hyla cinerea a signal that is nearly ignored when presented simultaneously with another, receives the majority of phonotaxis responses when presented in a leading or preceding temporal position [53] . This effect of timing has been shown across taxa [54] , [55] , including túngara frogs. Females prefer preceding calls and males compete to time their calls so that they precede others [56] . Although our data suggest that this preference for the leading signal is manifested in auditory grouping as well as during call choice, the reason for this exception in grouping responses is still unclear. This study reached three conclusions regarding auditory object formation in mate-searching frogs. When multiple sources create the potential for multiple auditory groups: túngara frogs use relative spatial separation to make grouping decisions; spatial acuity for grouping is not explained by spatial acuity for masking; and schema-based cues from call sequence can be used to include or exclude calls from auditory groups. These are important because they: reveal the perceptual mechanisms that enable females to assign sexual signals to males, a process inextricably linked to mate choice; and elucidate common cognitive processing that are shared by widely disparate taxa in solving similar problems. Subjects Females were collected in amplexus in Gamboa, Panama approximately 3 h after sunset in June 2007–2009. Animals were marked (toe clipped) to prevent retesting. All procedures were performed in accordance with the guidelines established by the Smithsonian Tropical Research Institute, the University of Texas and LSUHSC Animal Care and Use Committees. Experimental procedure The experimental procedure is the same as that used previously [30] , [31] . Phonotactic responses were measured to whines and chucks presented alone or in combination at various spatial separations. Each trial began by placing a gravid female P. pustulosus beneath a mesh cone (10 cm diameter) at the center of a circular array of 5 speakers on the floor of the sound chamber. Following 3 min of exposure to the stimuli, the cone was remotely removed allowing a subject to move freely while the stimuli continued to play. Using an infrared camera, we (minimum of 3 observers) recorded the position (in 5° intervals) at which females exited the full perimeter. Video of all trials was recorded to confirm measurements. A positive response was recorded only if the female crossed the perimeter of the array within 15 min. 'No-choice' trials were scored when females (1) failed to leave the 10 cm center circle in 5 min, (2) remained stationary for 2 min, or (3) remained within the perimeter for 15 min. To ensure that 'no-choice' scores were due to the stimuli and not a lack of female motivation, females exhibiting consecutive 'no-choice' responses were not tested again. Females were tested only once per stimulus. Subjects controlled their orientation with respect to the speakers at all times during the experiments (that is, in or out of the cone). Although this design differs from that with headphones or head holders in humans, it maintains the ethological relevance of the task, as females must not only determine sound source location, they must also walk to it. All trials were performed within 12 h of sunset under infrared illumination. Ambient temperature was ∼ 27°C. Within the natural range produced by males, the peak amplitude of all chucks was 6 dB re. whine amplitude (90 dB SPL re. 20 μPa; call amplitude at 50 cm [57] ). For each experiment, stimuli were presented in random order. Females remain responsive for up to ∼ 18 different stimulus presentations. Because the experiments here are comprised of >30 different stimuli, the experiments were run on three separate sample populations over three summers. Stimuli For consistency, the whine and chuck were the same as those used by Farris et al . [30] , [31] ( Fig. 1 ). These call components were those of an average call from Gamboa, where we collected females. The average was calculated from 14 acoustic variables from 250 complex calls of 50 males (five calls per male) [58] . Call period for all stimuli was 2 seconds. Stimuli were generated using an Audigy 2 ZS (Creative Labs) 7 channel sound card; amplified using Crown (XLS 202) amplifiers; and broadcast from Radioshack 4 inch broadband speakers (# 40–1040) speakers positioned along the perimeter of a 75 cm radius arc inside an Acoustic Systems sound chamber (2.75×1.83 m) lined with additional anechoic foam along the bottom 0.6 m of each wall (Sonex, 1.5 inch). Prior to each night's trials, the peak amplitude of the whine and chuck stimuli were calibrated using a 500 Hz tone, a GenRad 1982 sound level meter (Fast, linear weighting) and 0.5 inch microphone placed 3 cm above the floor of the arena at the center of the arc. To control for potential position effects and to reduce any phonotactic bias due to potential speaker variability, the broadcast orientation (in the array) was randomized. Furthermore, the speakers were switched three times during an experiment (after ∼ 7 females). Effect of relative spatial separation experiment Chucks cannot be produced by themselves due to morphological constraint [29] . Thus, whine-chuck spatial coherence is a potential cue for grouping. However, previous data showed that for a single whine and a single chuck, absolute spatial separation had very little effect on grouping: significant grouping occurred up to 135° whine-chuck separation [30] , [31] ( Fig. 1 ). With the addition of a second chuck, experiments here used 3 stimuli to test whether the relative whine-chuck separation affects grouping. Using the circular phonotaxis arena described above, a single whine was presented in natural sequence with two identical chucks that varied independently in spatial separation from the whine (0–180°). Because of the importance of spatial orientation in the acuity of auditory spatial processing [34] , two permutations were used. The first varied the relative whine-chuck spatial separation of the two chucks so that that they were on the same side of the whine. This means that when the whine is at 0° normal to the front of the frog the two chucks are lateralized in the same hemisphere. The second permutation used the same relative whine-chuck separations, but placed the chucks on opposite sides of the whine, allowing for tests of whether relative spatial cues are affected by lateralization. The direction of female phonotaxis (that is, the exit angle from the arena) was measured to test the null hypothesis that grouping is directed towards the chuck closest to the whine, showing that object formation results from comparisons between spatial separations. Spatial acuity of masking and grouping experiment The categorical grouping responses in experiment 1 (see results ) suggested that only one of the spatially separated chucks may be detected at a time, raising the possibility that there is high spatial acuity around a single chuck (see results ). Thus, different from the grouping task, this experiment examined the spatial resolution for chuck detection using a masking paradigm (cf. spatial release from masking). Here, a single whine and chuck were presented in the natural sequence at a constant 90° spatial separation, well within the grouping angle for single whines and chucks [30] , [31] . Band-limited (50 Hz–10 kHz; 98 dB/octave skirts) noise with the chuck's envelope structure (Hilbert transform [59] ) was presented simultaneously with the chuck from a third speaker. The bandwidth was chosen to encompass the spectrum of the entire chuck, as full spectrum chucks are more likely grouped than filtered ones [31] . The experiment measured the smallest chuck-noise separation which still enabled the conditional response to the chuck (that is, where the chuck was not masked and still grouped with the whine). Effect of relative sequence experiment The morphologically limited whine-then-chuck syntax provides a schema-based cue for grouping [29] . For example, chucks and whines with simultaneous onsets cannot be produced by the same male. Thus, this experiment used 3 stimuli: a whine and two chucks at equal spatial separation (90° re. whine). Relative to that of the whine, the timing of the two chucks is varied to test whether grouping is more likely for the chuck that was broadcast closest to the time of the natural sequence. Analysis Using females' exit angles from the circular arena, we employed both categorical and circular analyses to assess which stimuli elicited a conditional response to the chuck, an indication of perceptual group formation. For categorical analysis, exit angles were grouped into one of two categories. The first category included those responses in which females exited the perimeter and made contact with the speaker (a 20° arc; 13 cm). The second category included all other exit angles as well as those trials exhibiting 'no choice' responses. No choice responses, especially to the chuck alone are biologically relevant but cannot otherwise be included in the circular analyses below. A Fisher exact test assessed whether the number of responses in each category differed between stimulus conditions or expected response numbers generated by previous data [30] , [31] . For the circular analyses, the effect of chuck position on phonotactic direction was analyzed using three different tests. First, a Rayleigh test for circular uniformity tested whether exit angles were randomly distributed. Second, a V-test determined whether responses were localized at a particular exit angle [60] . The V-test, however, is most powerful when the distribution of exit angles is unimodal. Because phonotaxis is also directed to the whine in some trials, the V-test may lack resolution for smaller spatial separations. Thus, differences in mean exit angles between various broadcast conditions were analyzed using an additional method, the Watson-Williams test [60] with alpha correction for multiple comparisons. By comparing distributions of exit angles between different stimulus conditions, this test reveals whether the exit angles were affected by altering the stimuli. Whereas the V-test determines if phonotaxis is localized at a certain separation angle, the Watson-Williams test assesses whether the distribution is different from that for control broadcasts (for example, whine alone; whine and single chuck). Watson-Williams tests are not performed with distributions that are not different from random, however, as the mean of such a distribution will have 180° variance, causing the test to show that it has a similar mean to any other distribution. Unlike the categorical analysis, circular analyses were restricted to trials in which the females exited the perimeter, excluding 'no choice' responses. How to cite this article: Farris, H.E., & Ryan, M.J. Relative comparisons of call parameters enable auditory grouping in frogs. Nat. Commun. 2:410 doi: 10.1038/ncomms1417 (2011).